Generation and expansion of highly pure motor neuron progenitors from human pluripotent stem cells Human pluripotent stem cells (hPSCs) have opened new opportunities for understanding human development, modelling disease processes and developing new therapeutics. However, these applications are hindered by the low efficiency and heterogeneity of cell types, such as motorneurons (MNs), differentiated from hPSCs as well as our inability to maintain the potency of lineage-committed progenitors. Here by using a combination of small molecules that regulate multiple signalling pathways, we develop a method to guide human embryonic stem cells to a near-pure population (>95%) of motor neuron progenitors (MNPs) in 12 days, and an enriched population (>90%) of functionally mature MNs in an additional 16 days. More importantly, the MNPs can be expanded for at least five passages so that a single MNP can be amplified to 1 × 10 4 . This method is reproducible in human-induced pluripotent stem cells and is applied to model MN-degenerative diseases and in proof-of-principle drug-screening assays. Human pluripotent stem cells (PSCs), including embryonic stem cells (ESCs) and induced pluripotent stem cells (iPSCs), offer a new model system to explore early human development and dissect disease processes, as well as an opportunity to devise therapeutics [1] , [2] , [3] . A critical requirement for achieving these potentials is directed differentiation of hPSCs to target cell types. Substantial progress has been made in guiding hPSCs to major cell lineages, including blood, cardiac and neural cells [4] , [5] , [6] . Nevertheless, generation of highly pure cellular populations in large quantities, which are often necessary for biochemical analysis, disease modelling and clinical application, has not been readily achieved. In particular, it is often desired to obtain functionally specialized subtypes of cells from hPSCs; however, these populations represent only a tiny fraction of the cells in a normal tissue/organ of our body. Such a need poses critical challenges to the stem cell field. Spinal motor neurons (MNs) are a highly specialized type of neurons that reside in the ventral horns and project axons to muscles to control their movement. Degeneration of MNs is implicated in a number of devastating diseases, including spinal muscular atrophy (SMA), amyotrophic lateral sclerosis (ALS), Charcot-Marie-Tooth and poliomyelitis disease. The above disease iPSCs have been generated from patients and attempts have been made to identify disease-related phenotypes and to dissect out the underlying mechanisms before embarking on drug discovery [7] , [8] , [9] , [10] . However, these efforts are hindered by our inability to produce pure or highly enriched MNs with consistent quality. A number of protocols have been developed, including neural progenitor induction followed by neural patterning by retinoic acid (RA) and sonic hedgehog (SHH) [11] , [12] , neural progenitor induction followed by genetic manipulations using adenovirus-mediated gene delivery [13] and differentiation of MNs with above methods followed by sorting with green fluorescent protein (GFP) labelling under the MNX1 (also known as HB9 ) promoter [14] . These differentiation protocols are tedious, time-consuming (1–2 months) and are of low efficiencies (30–70%) unless by sorting (90%). Furthermore, PSC-derived neurons in vitro , including MNs, are often immature, making it difficult to reveal disease phenotypes that are manifested in functionally mature cells. Hence, there is a critical need to develop new methods that enable generation of highly pure and functionally mature MNs with consistent quality and in a short time. By using a combination of small molecules in a chemical defined neural medium, we have guided hPSCs to a near-pure population of OLIG2 + MNPs in 12 days, and a highly enriched population of functionally mature MNs (>90%) in another 16 days by the use of a Notch inhibitor. Furthermore, our approach enables expanding a single MNP to 1 × 10 4 MNPs, producing a large quantity (5 × 10 5 ) of consistent MNs from a single stem cell. MNs generated by this method display molecular phenotypes of SMA and ALS, and can be readily adapted to screening platforms, as illustrated by our luciferase-based axonal length assay using ALS patient MNs. Generation of highly pure MNPs by a small-molecule cocktail Specification of MNPs follows serial and overlapping developmental steps: neural induction as well as caudalization and ventralization of neuroepithelial progenitors (NEPs) [11] , [15] . In the presence of small molecules, SB431542 (SB, inhibitor of activin-nodal signalling, 2 μM) and DMH1 (DMH, inhibitor of bone morphogenetic protein signalling, 2 μM) [16] , [17] , hESCs (line H9) were induced to NEPs, with 77±9% of the total differentiated cells being SOX1 + ( Fig. 1a,b ). Activation of WNT by a small molecular agonist CHIR99021 (CHIR) has been shown to promote neural induction and potentially also neuroepithelial proliferation [18] , [19] . Under the treatment of 3 μM CHIR together with 2 μM SB+2 μM DMH for 6 days, nearly all the differentiated cells were SOX1 + NEPs (>98%; Fig. 1a,b ). CHIR not only augmented the efficiency of neural induction but also increased the yield of SOX1 + NEPs by 2.8-fold ( Fig. 1b ). Wnt activation (by CHIR) often induces a caudal fate of neural progenitors [20] . Indeed, CHIR-induced NEPs showed a caudal identity with HOXA3 expression. In contrast, NEPs induced by SB+DMH (without CHIR) exhibited a rostral identity with OTX2 expression ( Fig. 1b ). Therefore, treatment of CHIR+SB+DMH combines the steps of induction and caudalization of NEPs, representing a chemically defined, single-step method for obtaining homogenous caudal NEPs from hPSCs. 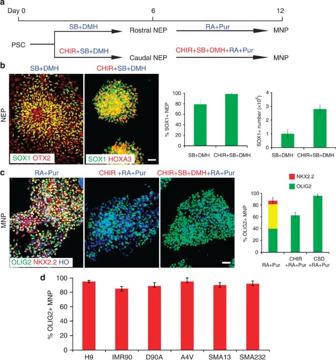Figure 1: Generation of highly pure population of MNPs from hPSCs. (a) Schematics showing the time course and small-molecule cocktail for hPSC differentiation into MNPs. (b) Representative images ofSOX1+NEPs after 6 days of culture in CHIR+SB+DMH versus SB+DMH condition. The regional identity (OTX2+ versusHOXA3+) were stained. Scale bars, 50 μm. Quantification ofSOX1+ NEP percentage and number is shown on right (>500 cells from random fields were manually counted in each condition). The bar graph shows the mean±s.d. (n=3 in each condition). (c) Representative images of pure MNPs on Day12 under different conditions, which expressOLIG2(green) but notNKX2.2(red). Scale bars, 50 μm. Quantification ofOLIG2+,NKX2.2+ andOLIG2+/NKX2.2+ cells is shown on right (>500 cells from random fields were manually counted in each condition). The bar graph shows the mean±s.d. (n=3 in each condition). (d) The efficiency ofOLIG2+MNP differentiation from multiple hPSC lines (>500 cells from random fields were manually counted in each cell line). The bar graph shows the mean±s.d. (n=3 in each cell line). Figure 1: Generation of highly pure population of MNPs from hPSCs. ( a ) Schematics showing the time course and small-molecule cocktail for hPSC differentiation into MNPs. ( b ) Representative images of SOX1 +NEPs after 6 days of culture in CHIR+SB+DMH versus SB+DMH condition. The regional identity ( OTX2 + versus HOXA3 +) were stained. Scale bars, 50 μm. Quantification of SOX1 + NEP percentage and number is shown on right (>500 cells from random fields were manually counted in each condition). The bar graph shows the mean±s.d. ( n =3 in each condition). ( c ) Representative images of pure MNPs on Day12 under different conditions, which express OLIG2 (green) but not NKX2.2 (red). Scale bars, 50 μm. Quantification of OLIG2 +, NKX2.2 + and OLIG2 +/ NKX2.2 + cells is shown on right (>500 cells from random fields were manually counted in each condition). The bar graph shows the mean±s.d. ( n =3 in each condition). ( d ) The efficiency of OLIG2 + MNP differentiation from multiple hPSC lines (>500 cells from random fields were manually counted in each cell line). The bar graph shows the mean±s.d. ( n =3 in each cell line). Full size image The next step is to specify OLIG2 + MNPs by mimicking the ventralization of NEPs in vivo . By exposing the CHIR+SB+DMH-induced caudal-like NEPs to RA (0.1 μM) and Pur (Purmorphamine, SHH signalling agonist, 1 μM) for 6 days, which was identified in our previous study [21] , we obtained 81±9% OLIG2 -expressing neural progenitors ( Fig. 1c ). However, ~40% OLIG2 + cells co-expressed with NKX2.2 , another ventral spinal cord marker ( Fig. 1c ). During neural development, OLIG2 and NKX2.2 are initially induced in a common pool of progenitors that ultimately segregate into unique territories, giving rise to distinct OLIG2 + MNPs and NKX2.2 + interneuron progenitors [22] . WNT signalling plays a critical role in this segregation [23] . We thus added WNT agonist CHIR in combination with RA and Pur. Under the treatment of CHIR+RA+Pur for 6 days, NKX2.2 expression was completely repressed in the culture, but OLIG2 -expressing population was also decreased to 62±5% ( Fig. 1c ). We reasoned that WNT signalling may elevate the threshold of SHH signalling necessary to induce OLIG2 expression. However, at the increased concentration, SHH agonist Pur became toxic to the NEPs. We thus took an alternative approach to decrease the threshold of SHH signalling by repressing the dorsalizing molecule of the spinal cord, BMP signalling. Addition of dual inhibitors SB and DMH in combination with CHIR+RA+Pur significantly increased OLIG2 + / NKX2.2 − cell population ( Fig. 1c ). By serial titration of Pur and CHIR in combination with RA, SB and DMH ( Supplementary Fig. 1 ), we found that treatment with 1 μM CHIR, 2 μM SB, 2 μM DMH, 0.1 μM RA and 0.5 μM Pur for 6 days resulted in a robust population of OLIG2 + MNPs (95±3%), among which few (<0.5%) OLIG2/NKX2.2 double-positive cells were found ( Fig. 1c ). Our protocol for OLIG2+ MNP specification is highly reproducible in multiple different hPSC lines, including normal iPSC line IMR90, ALS iPSC lines SOD1-D90A and SOD1-A4V, and SMA iPSC lines SMA13 and SMA232 ( Fig. 1d ). Under the treatment of CHIR+SB+DMH for 6 days and CHIR+SB+DMH+RA+Pur for another 6 days, all the hPSC lines generated more than 90% OLIG2 + MNPs. Thus, coordinated specification and patterning of neuroepithelia by small molecules lead to robust generation of pure population of region-specific MNPs. MNPs can be expanded to large numbers Developmentally, OLIG2 + MNPs are present transiently and they transition to other neuronal (interneuron) and glial (oligodendrocyte) lineages after generation of MNs. For cellular and biochemical analyses, it is crucial to expand the MNPs without losing their ability to produce MNs, which has not been achieved. Since the CHIR+SB+DMH+RA+Pur condition is highly efficient in specifying and generating MNPs, we asked whether the condition could expand the OLIG2 + MNPs in a continuously dividing state. We first examined whether RA and Pur are required for maintaining OLIG2 expression. The MNPs were passaged weekly under the CHIR+SB+DMH1 condition with or without Pur or RA+Pur. After two passages, OLIG2 + MNPs were decreased to 35±5% in the control group (without Pur and RA), to 62±5% in Pur group, and a large population of NKX2.2 + cells appeared in these two groups. In the RA+Pur group, OLIG2+ MNPs were maintained at 91±3% with rare NKX2.2 + cells ( Fig. 2a ). Therefore, RA and Pur are required for maintaining the identity of MNPs. 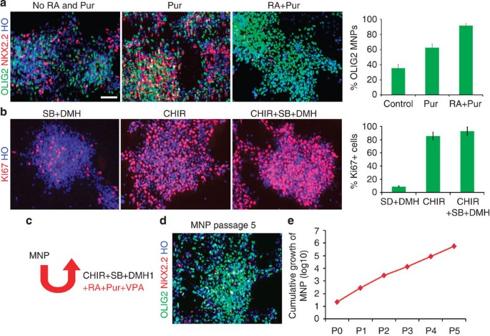Figure 2: Expansion ofOLIG2+MNPs. (a) Representative images of pureOLIG2+ (green)/NKX2.2+(red) MNPs maintained under different conditions. Scale bars, 50 μm. Quantification ofOLIG2+/NKX2.2−cells is shown on right (>500 cells from random fields were manually counted in each condition). The bar graph shows the mean±s.d. (n=3 in each condition). (b) Representative images ofKi67+ (red) proliferating progenitors maintained under different conditions. Scale bars, 50 μm. Quantification ofKi67+cells is shown on right (>500 cells from random fields were manually counted in each condition). The bar graph shows the mean±s.d. (n=3 in each condition). (c) Schematics showing the expansion of MNPs with the combination of small molecules. (d) Representative images of MNPs expanded for at least five passages, yet maintained the OLIG2 (green) expression. (e) Cumulative hPSC-derived MNP counts over five passages (passages denoted p1–p5). One six-well of cells were manually counted in each passage, and total cell numbers were calculated by time passage ratio. Figure 2: Expansion of OLIG2 + MNPs. ( a ) Representative images of pure OLIG2 + (green)/ NKX2.2 + (red) MNPs maintained under different conditions. Scale bars, 50 μm. Quantification of OLIG2 +/ NKX2.2− cells is shown on right (>500 cells from random fields were manually counted in each condition). The bar graph shows the mean±s.d. ( n =3 in each condition). ( b ) Representative images of Ki67 + (red) proliferating progenitors maintained under different conditions. Scale bars, 50 μm. Quantification of Ki67 + cells is shown on right (>500 cells from random fields were manually counted in each condition). The bar graph shows the mean±s.d. ( n =3 in each condition). ( c ) Schematics showing the expansion of MNPs with the combination of small molecules. ( d ) Representative images of MNPs expanded for at least five passages, yet maintained the OLIG2 (green) expression. ( e ) Cumulative hPSC-derived MNP counts over five passages (passages denoted p1–p5). One six-well of cells were manually counted in each passage, and total cell numbers were calculated by time passage ratio. Full size image We then examined whether CHIR, SB and DMH are required for maintaining cell proliferation. The MNPs were passaged under the RA+Pur condition and divided into three groups: SB+DMH treatment group, CHIR treatment group and CHIR+SB+DMH treatment group. After two passages, the cell population expressing Ki67, a cell proliferation marker, was at less than 8%, 81±6% and 92±4% in the SB+DMH group, the CHIR group and the CHIR+SB+DMH group, respectively ( Fig. 2b ). Therefore, CHIR+SB+DMH are required for maintaining the proliferation of MNPs at the maximum level. When the MNPs were expanded in the same media (CHIR+SB+DMH+RA+Pur) for longer than two passages, the OLIG2 -expressing MNP population decreased with a concomitant appearance of MNX1 expressing MNs, suggesting that some MNPs have exited cell cycle and differentiated to neurons. We reasoned that this is likely due to the neurogenic effect of RA. It was known that valproic acid (VPA), a histone deacetylase inhibitor, can repress neurogenesis by indirectly activating Notch signalling [24] . We thus added VPA to the culture system. Under this culture condition, the MNPs were expanded for at least five passages, yet maintained OLIG2 expression at 82±9% ( Fig. 2d ). Further culturing under this condition resulted in a gradual decrease in OLIG2 + cell population and increase in NKX2.2 + cell population, suggesting a need of alternative strategy for an even longer-term expansion. Nevertheless, continual expansion of MNPs for five passages allows amplification of a single MNP to 1 × 10 4 MNPs, translating to the generation of >5 × 10 5 MNPs from a single hPSC ( Fig. 2e ). Furthermore, these MNPs can be frozen and thawed under regular condition with over 90% recovery. MNPs differentiate into an enriched population of functional MNs To determine the differentiation of expanded MNPs, we withdrew CHIR+SB+DMH, increased RA concentration (0.5 μM) and reduced Pur (0.1 μM). After 6 days, nearly all the MNPs differentiated into MNs, as evidenced by expression of MNX1 (90±9%) or ISL1 (95±3%; Fig. 3a,b ). Further culture on Matrigel or astrocyte feeders for 2 weeks resulted in generation of more mature MNs that expressed CHAT , although the CHAT + MN population (47±9%) was substantially lower than the MNX1 + MNPs. We reasoned that the lower population of CHAT + mature MNs may be due to proliferation of the small number of neural precursors and their subsequent differentiation to other neuronal types via lateral inhibition of NOTCH signalling [25] . To overcome this inefficiency of MN maturation, we applied Compound E (Cpd E), a NOTCH signalling inhibitor in the MN culture. Cpd E treatment for 10 days resulted in a near homogenous MAP2 + mature neuronal cultures without any proliferating cells (Ki67 + ), and ~91±6% of MAP2 + neurons expressed CHAT ( Fig. 3a,b ). These CHAT+MNs were electrophysiologically active, as defined by their ability to elicit action potentials in response to depolarizing current injection in current-clamp recordings ( Supplementary Fig. 2 ). Therefore, Cpd E not only increases the mature MN population but also substantially shortens the maturation process. 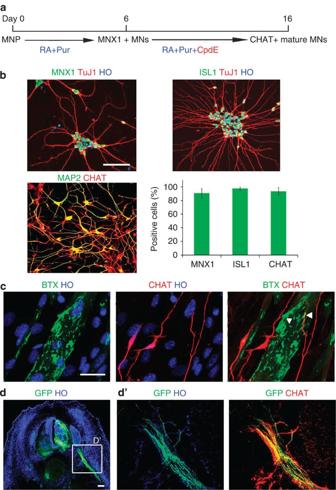Figure 3: MNPs differentiate into enriched functional MNs. (a) Schematics showing the time course and small-molecule cocktail for MNP differentiation into mature MNs (>500 cells from random fields were manually counted in each condition). The bar graph shows the mean±s.d. (n=3 in group). (b) Representative images of MNs showingMNX1+,ISL1+(green) andCHAT+(red) on. Scale bars, 50 μm. Quantification ofMNX1+,ISL1+andCHAT+is shown (c) MNs, stained with the CHAT antibody (red), formed neuromuscular junctions, labelled with bungarotoxin (BTX, green), when co-cultured with myotubes. Scale bars, 100 μm. (d) Representative image of xenotransplantation of GFP-labelled human MNs into a developing chicken embryo. Scale bars, 50 μm. (d′) Magnification of the field showing that human MN axons (GFP+/CHAT+) projected ventrally through the ventral roots. Figure 3: MNPs differentiate into enriched functional MNs. ( a ) Schematics showing the time course and small-molecule cocktail for MNP differentiation into mature MNs (>500 cells from random fields were manually counted in each condition). The bar graph shows the mean±s.d. ( n =3 in group). ( b ) Representative images of MNs showing MNX1 + , ISL1 + (green) and CHAT + (red) on. Scale bars, 50 μm. Quantification of MNX1 + , ISL1 + and CHAT + is shown ( c ) MNs, stained with the CHAT antibody (red), formed neuromuscular junctions, labelled with bungarotoxin (BTX, green), when co-cultured with myotubes. Scale bars, 100 μm. ( d ) Representative image of xenotransplantation of GFP-labelled human MNs into a developing chicken embryo. Scale bars, 50 μm. ( d ′) Magnification of the field showing that human MN axons (GFP + / CHAT + ) projected ventrally through the ventral roots. Full size image To determine whether the Cpd E-accelerated MNs are functional, we co-cultured the MNs with differentiated myotubes from mouse C2C12 cells. After 10 days of co-culture, we observed aggregated BTX + acetylcholine receptors on myotubes and their overlapping with CHAT + neurites ( Fig. 3c ), suggesting the formation of neuromuscular junctions. To study the ability of MNs to project axons towards the muscle targets, Cpd E-treated MNs were transplanted in ovo into the lesion neural tube of chicken embryos at HH stage15–16. Transplanted embryos showed successful engraftment of human MNs (as marked by GFP expression) into the ventral horn ( Fig. 3d ). Importantly, we observed GFP-labelled human MN axons ( CHAT + ) projected ventrally through the ventral roots and along the peripheral nerves of the host ( Fig. 3d’ ). These data indicate that mature MNs generated by the Cpd E treatment exhibit proper functions. Use of enriched MNs for disease modelling and screening Most neurodegenerative diseases, such as SMA and ALS, preferentially affect one type of neurons such as MNs. Genetically linked disorders, including SMA and ALS, may lead to changes in gene dosage at less than 50%. Hence, it will be technically difficult to discern changes in gene expression if the population of disease target cells is not highly enriched. To determine the utility of the MNs generated with the above method, we measured the expression of genes that are known to be altered in SMA and ALS. In this analysis, we generated spinal non-MNs from the same iPSCs as a control by replacing Pur with Cyclopamine to block SHH signalling ( Supplementary Fig. 3a ). Under RA and Cyclopamine treatment for 6 days, the induced spinal neural precursors were void of OLIG2 expression, and the differentiated neurons were void of MNX1 and CHAT expression, but with GABA (γ-aminobutyric acid) expression ( Supplementary Fig. 3b,c ). Using these highly enriched MNs and GABA neurons, we found that the mRNA of survival motor neuron ( SMN ) was decreased in both MNs and GABA neurons that were derived from SMA patients as compared with those from non-SMA iPSCs ( Fig. 4a ). This is consistent with the fact that SMN mutations affect all cell types. Interestingly, we found that MNs exhibited even lower (38±4%) SMN than that in GABA neurons (60±6%; Fig. 4a ), again consistent with a previous report that MNs express markedly lower levels of full-length SMN transcripts from the SMN2 gene than do other cells in the spinal cord [26] . Similarly, in ALS caused by mutations in the superoxide dismutase ( SOD1 ) gene, MNs display neurofilament (NF) aggregation that is attributed to the decreased level of light polypeptide neurofilament ( NEFL ) [9] , we found a 45±4% reduction of NEFL mRNA in D90A MNs, but not GABA neurons, when compared with genetically corrected (D90D) MNs and GABA neurons ( Fig. 4b ). Together, these data indicate that the enriched MNs generated from patient iPSCs using our new method enable identification of disease-related phenotypes. 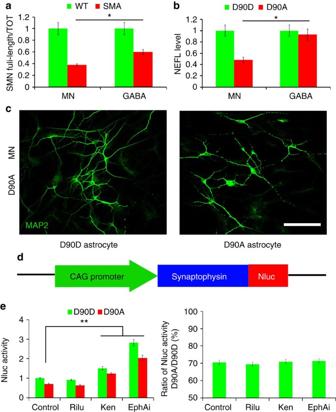Figure 4: Enriched MNs for disease modelling and screening. (a) The qPCR quantification of the ratio of full-length SMN versus total SMN in wild-type (WT) and SMA disease MNs, GABA neurons. The bar graph shows the mean±s.e.m. (*P<0.05,t-test,n=3 in each group). (b) The qPCR quantification of theNEFLmRNA level in ALS (D90A) and corrected (D90D) MNs, GABA neurons. The bar graph shows the mean±s.e.m. (*P<0.05,t-test,n=3 in each group). (c) Representative image of ALS (D90A) MNs when culturing on ALS (D90A) astrocytes and corrected (D90D) astrocytes, which showed neurite fragmentation and reduced neurite length. Scale bars, 50 μm. (d) Schematics of SYP-Nluc reporter. (e) Quantification of Nluc activity (left panel) and ratio (right panel) of SYP-Nluc reporter MNs on ALS (D90A) and corrected (D90D) astrocytes, when comparing between the control, Riluzole (Rilu), Kenpaullone (Ken) and EphA inhibitor (EphAi) groups. The bar graph shows the mean±s.e.m. (**P<0.01, Tukey’s test,n=8 in each group). Figure 4: Enriched MNs for disease modelling and screening. ( a ) The qPCR quantification of the ratio of full-length SMN versus total SMN in wild-type (WT) and SMA disease MNs, GABA neurons. The bar graph shows the mean±s.e.m. (* P <0.05, t -test, n =3 in each group). ( b ) The qPCR quantification of the NEFL mRNA level in ALS (D90A) and corrected (D90D) MNs, GABA neurons. The bar graph shows the mean±s.e.m. (* P <0.05, t -test, n =3 in each group). ( c ) Representative image of ALS (D90A) MNs when culturing on ALS (D90A) astrocytes and corrected (D90D) astrocytes, which showed neurite fragmentation and reduced neurite length. Scale bars, 50 μm. ( d ) Schematics of SYP-Nluc reporter. ( e ) Quantification of Nluc activity (left panel) and ratio (right panel) of SYP-Nluc reporter MNs on ALS (D90A) and corrected (D90D) astrocytes, when comparing between the control, Riluzole (Rilu), Kenpaullone (Ken) and EphA inhibitor (EphAi) groups. The bar graph shows the mean±s.e.m. (** P <0.01, Tukey’s test, n =8 in each group). Full size image Our ability to generate large quantity of consistent MNs offers an opportunity for building high-throughput screening platforms for MN diseases. In ALS, astrocytes enhance disease progression by promoting axonal degeneration and MN death [27] , [28] , [29] . Indeed, when ALS iPSC-derived MNs were grown on top of ALS (D90A SOD1) or genetically corrected (D90D SOD1 ) astrocytes ( Supplementary Fig. 4 ) in a medium that lacks neurotrophic factors, MNs began to show neurite fragmentation with reduced neurite length on D90A but not D90D astrocytes on Day 10 ( Fig. 4c ). To enable automated measurement of neurite length for high-throughput screening, we established a reporter iPSC line (from D90A SOD1 ) with a luciferase reporter NanoLuc (Nluc) fused with SYNAPTOPHYSIN (SYP; Fig. 4d ), a synaptic vesicle glycoprotein, which targets the Nluc reporter to the axonal membrane, not the cytoplasm [30] . We first established the linear relationship between Nluc expression and MN numbers by measuring luciferase activity of cultures 10 days after plating different numbers of SYP-Nluc-expressing MNs (1,250, 2,500, 5,000, 10,000 and 20,000 cells) on astrocytes ( Supplementary Fig. 5a ). We then tested whether the Nluc reporter activity is correlated with the reduced axonal length. Same numbers of SYP-Nluc-expressing MNs were plated on D90D and D90A astrocytes, and the Nluc activity was detected on Day 10. The Nluc activity on D90A astrocytes was significantly decreased to 70.5±2.7%, comparing with the D90D astrocyte group ( Supplementary Fig. 5b ). Next, we exposed the co-cultures to three compounds, Riluzole (Rilu) [31] , the only approved drug for ALS, as well as Kenpaullone (Ken) and EphA inhibitor (EphAi) that are known to rescue axonal degeneration in ALS cell models [32] , [33] . Riluzole had no effect on Nluc activity. Ken and EphAi increased the Nluc activity to 1.5- and 2.8-fold, respectively, in both D90A and D90D groups ( Fig. 4e ), indicating that they increased axonal length. However, Ken and EphAi did not specifically rescue the axonal length of MNs induced by ALS astrocytes, as the ratio of Nluc activity on D90A astrocytes versus D90D astrocytes remained at 70% ( Fig. 4e ). These results provide a proof-of-principle for the use of our enriched, patient-derived MNs for drug screening and suggest its potential for identifying disease-specific targets. We have developed a strategy for guiding hPSCs to a near-pure population of OLIG2 + MNPs in 12 days by coordinating signalling pathways using small molecules, and subsequently a highly enriched population of functionally mature MNs (>90%) in another 16 days by the use of a Notch inhibitor. Furthermore, we have devised a method to expand a single MNP to 1 × 10 4 MNPs, enabling production of a large quantity (5 × 10 5 ) of consistent MNs from a single stem cell. Our approach enables presentation of disease phenotypes and building of screening platforms, as illustrated by our luciferase-based axonal length assay using ALS patient MNs. Compared with previous methods, our method has two critical improvements. The first is the application of WNT agonist during MNP differentiation. WNT signalling is a more efficient pathway to caudalize neural progenitors [20] . Thus, the combination of WNT activator with dual SMAD inhibitors induced homogenous caudal NEPs from hPSCs. Most importantly, WNT signalling plays a critical role in MNP specification. All previous methods used RA and SHH to induce OLIG2 + MNPs without examining other ventral spinal markers, especially co-expression of NKX2.2 . We showed here that RA and SHH condition generated mixed ventral progenitors with a large population of cells that co-express OLIG2 and NKX2.2 . During spinal cord development, OLIG2 and NKX2.2 are initially induced in a common pool of progenitors that ultimately segregate into unique territories, giving rise to distinct OLIG2 + MNPs (pMN domain) and NKX2.2 + interneuron progenitors (p3 domain) [22] . Without segregation, NKX2.2 could interfere with the differentiation of OLIG2 + progenitors to MNX1 + MNs, which is one of the reasons why some previous methods induced a high percentage of OLIG2 + progenitors, but ended with a small population of MNX1 + MNs. WNT signalling was reported to selectively oppose SHH-mediated induction of NKX2.2, but have little effect on OLIG2, and thereby establish their distinct expression domains in cooperation with graded SHH signalling [23] . As WNT elevates the strength of SHH signalling to induce OLIG2 expression, the two inhibitors of dorsalizing BMP signalling were also included. Therefore, our method of combining with small molecules regulating WNT, SHH, RA and BMP signallings closely mimics the cooperation of these signallings in the spinal cord development in vivo to specify the region-specific OLIG2 + MNPs. Recently Maury et al. [34] also applied WNT agonist CHIR in the generation of MNs from hPSCs. However, the treatment condition under which CHIR was applied is different, and the NKX2.2-expressing cell population was not examined. It will be interesting to compare two approaches in specifying MNPs. The second improvement is the application of a NOTCH inhibitor during MN maturation. Lateral inhibition mediated by NOTCH signalling is an intrinsic mechanism to guide orderly transition of mitotically active precursors into different types of post-mitotic neurons and glia at different stages [25] . The treatment with NOTCH inhibitor Cpd E in our method synchronizes the differentiation of OLIG2 + MNPs to generate homogenous mature MNs without mixing with any other neural cells. With these two improvements, our method robustly generates almost homogenous mature MNs, which exhibit functional properties, including formation of neuromuscular junctions when co-cultured with skeletal muscle cells and projection of axons towards muscles when grafted into the developing chick spinal cord. More significantly, the MNs derived from disease iPSCs by our method exhibit the MN-specific molecular phenotypes, including downregulation of full-length SMN in SMA and downregulation of the NEFL level in ALS, which would be nearly impossible to detect with previous methods that only generate a small population of MN in the mixed culture. A large quantity of consistent target cells, such as mature MNs, is necessary for high-throughput screening. In general, lineage-committed progenitors can be expanded, but quickly lose their differentiation potency. For example, OLIG2 + MNPs can be expanded with fibroblast growth factor and/or epidermal growth factor, but quickly lose the potency of MN differentiation into two passages. Several recent reports described the expansion of neural progenitors with small molecules of WNT and/or SHH signallings [18] , [35] . However, as shown in this study ( Fig. 2a ), their ability to maintain MN potential is still significantly diminished during cell passages compared with our method. Our method can expand MNPs for at least five passages to amplify a single MNP to 1 × 10 4 MNPs, or generate 5 × 10 5 MNs from single hPSC. This provides a sufficient cell source for high-throughput drug screening, as shown in our screening platform for MN axonal degeneration. In summary, our new method enables the generation of large quantities of MNs with consistency and high purity, providing a basis for modelling MN diseases in vitro and for drug discovery. hPSCs The human PSC lines used in this study are listed in Supplementary Table 1 . Fibroblasts from a 50-year-old female ALS patient carrying the D90A SOD1 mutation (ND29149, Coriell Institute, coriell.org), a 3-year-old male SMA patient (GM03813, Coriell Institute) and a 7-month-old SMA patient (GM00232, Coriell Institute) were reprogrammed using the non-integrating Sendai virus as described [36] to established iPSC lines ALS-D90A, SMA13 and SMA232. The D90D iPSC line was established by correcting the D90A SOD1 mutation in ALS-D90A lines using TALEN technology [9] . A4V SOD1 mutant ALS iPSC line, established with retrovirus, was obtained from Coriell (ND35671). Human ESC line H9 (WA09 line, NIH registry 0046) and normal iPSC line IMR90-4 were obtained from WiCell. All the PSCs were cultured on irradiated mouse embryonic fibroblasts as described in the standard protocol http://www.wicell.org . MNP specification and MN differentiation To generate MNPs, hPSCs were dissociated with Dispase (1 mg ml −1 ) and split 1:6 on irradiated mouse embryonic fibroblasts or Matrigel-coated plates. On the following day, the PSC medium was replaced with a chemically defined neural medium, including DMEM/F12, Neurobasal medium at 1:1, 0.5 × N2, 0.5 × B27, 0.1 mM ascorbic acid (Santa Cruz), 1 × Glutamax and 1 × penicillin/streptomycin (all others from Invitrogen). CHIR99021 (3 μM, Torcris), 2 μM DMH1 (Torcris) and 2 μM SB431542 (Stemgent) were added in the medium. The culture medium was changed every other day. Human PSCs maintained under this condition for 6 days were induced into NEP cells. The NEP cells were then dissociated with Dispase (1 mg ml −1 ) and split at 1:6 with the same medium described above. RA (0.1 μM, Stemgent) and 0.5 μM Pur (Stemgent) were added in combination with 1 μM CHIR99021, 2 μM DMH1 and 2 μM SB431542. The medium was changed every other day. NEP cells maintained under this condition for 6 days differentiated into OLIG2+ MNPs. The OLIG2 + MNPs were expanded with the same medium containing 3 μM CHIR99021, 2 μM DMH1, 2 μM SB431542, 0.1 μM RA, 0.5 μM Pur and 0.5 mM VPA (Stemgent), and split 1:6 once a week with Dispase (1 mg ml −1 ). OLIG2 + MNPs were frozen with the regular frozen medium (DMEM/F12, 10% fetal bovine serum and 10% DMSO) in liquid nitrogen, and cultured again in expansion medium after thawing. To induce MN differentiation, OLIG2 + MNPs were dissociated with Dispase (1 mg ml −1 ) and cultured in suspension in the above neural medium with 0.5 μM RA and 0.1 μM Pur. The medium was changed every other day. OLIG2 + MNPs under this condition for 6 days differentiated into MNX1 + MNs. The MNX1 + MNs were then dissociated with Accumax (eBioscience) into single cells and plated on Matrigel-coated plates or on astrocytes. The MNX1 + MNs were cultured with 0.5 μM RA, 0.1 μM Pur and 0.1 μM Compound E (Calbiochem) for 10 days to mature into CHAT + MNs. Insulin-like growth factor 1, brain-derived neurotrophic factor and ciliary neurotrophic factor (all from R&D, 10 ng ml −1 each) were added if MNs were plated at low density. For identifying MN disease phenotypes, SMA and ALS MNs were cultured without these neurotrophic factors. Functional analysis of mature MNs Whole-cell patch-clamp recordings were performed on iPSC-derived CHAT + neurons on Day28 after iPSC differentiation. Briefly, neurons were held at −70 mV to record Na+/K+ channel activities, and at 0 mV to record spontaneous release. For recording action potentials, cells were held at 0 pA with the current-clamp model and the steps of currents from +0 pA were injected into cells by the holding electrode. The bath solution consisted of 127 mM NaCl, 1.2 mM KH2PO4, 1.9 mM KCl, 26 mM NaHCO 3 , 2.2 mM CaCl 2 , 1.4 mM MgSO 4 , 10 mM glucose, 290 mM mOsm and 95% O 2 /5% CO 2 . Recording pipettes were filled with an intracellular solution containing 20 mM KCl, 121 mM K+−gluconate, 10 mM Na+−HEPES, 10 mM BAPTA, 4 mM Mg 2 +−ATP pH 7.2 and 290 mOsm. An Olympus BX51WI microscope was used to visualize neurons. A MultiClamp 700B amplifer (Axon Instruments, Molecular Devices, Sunnyvale, CA, USA) was used to investigate the voltage clamp and current-clamp recordings. Signals were filtered at 4 kHZ and sampled at 100 kHz using a Digidata 1322A analogue-digital converter (Axon Instruments). Data were analysed with pClamp 9.0 (Axon Instruments). Capacitance and series resistance were compensated by 50–80% using an amplifier circuitry. To examine neuromuscular junction formation, C2C12 cells were seeded on Matrigel-coated plate in DMEM with 10% FBS, and then were induced to form myotube by switching to DMEM containing 2% FBS. On Day 18 MNX1 + MNs derived from hPSCs were plated on myotubes and cultured in maturation condition for 7 days, after which the neuromuscular synapses were visualized using CHAT and BTX staining. To perform transplantations, Day 18 MNX1 + MN spheres were triturated with a 1- ml pipette tip five to seven times and treated with Cpd E for 24 h. Transplantation was performed as previously described [15] . Briefly, after a small suction, lesion at the prospective intraspinal site was created in a chick embryo at stage 15–18 at somites 15–20, and MN spheres were loaded into a hand-held microinjector and placed into the lesion. After 6 days, the chicks were killed, fixed with 4% paraformaldehyde for 2 h at 4 °C and neurite outgrowth was accessed by cutting 30-μm sections of the spinal cord near the injected site. qPCR analysis Total RNAs were isolated with the RNeasy Plus Mini Kit (Qiagen) according to the manufacturer’s instructions. For quantitative PCR (qPCR), cDNA was synthesized from 1 μg total RNAs using iScript reverse transcription supermix (Bio-Rad). qPCR was performed using iTaq Universal SYBR Green Supermix (Bio-Rad). GAPDH gene was used as internal control to equalize cDNA. The following primers were used in this study: full-length SMN, forward-5′-CACCACCTCCCATATGTCCAGATT-3′, reverse-5′-GAATGTGAGCACCTTCCTTCTTT-3′; total SMN, forward-5′-ATGAGCTGTGAGAAGGGTGTTG-3′, reverse-5′-TTGCCACATACGCCTCACATAC-3′; NEFL, forward-5′-TTTCACTCTTTGTGGTCCTCA-3′, reverse-5′-AGACCCTGGAAATCGAAGC-3′; GAPDH, forward-5′-CTCTCTGCTCCTCCTGTTCGAC-3′ and reverse-5′-TGAGCGATGTGGCTCGGCT-3′. Immunostaining and microscopy Immunohistochemical staining was performed according to Zhang et al. (2001) [37] . The following primary antibodies were used: SOX1 (gIgG 1:1,000, R&D), OTX2 (mIgG, 1:2,000, DSHB), HOXA3 (mIgG 1:1,000, R&D), OLIG2 (rIgG 1:500, Chemicon), NKX2.2 (mIgG 1:100, DSHB), Ki67 (rIgG 1:200, Chemicon), MNX1 (mIgG 1:50, DSHB), ISL1 (mIgG 1:1,000, DSHB), TUJ1 (rIgG 1:5,000, Covance), CHAT (gIgG 1:300, Chemicon), MAP2 (mIgG 1:1,000, Chemicon), GABA (mIgG 1:1,000, Chemicon) and FoxP1 (rIgG, 1:1,000, Chemicon). MN-astrocyte co-culture and luciferase assay The luciferase reporter Nluc was obtained from Promega. The SYP-Nluc reporter iPSC line was established by inserting SYP-Nluc fusion reporter in the AAVS1 site by the TALEN technology [38] . Six-month astrocytes were differentiated from the isogenic iPSC lines D90D and D90A by the protocol established in our laboratory [39] . The astrocytes were plated at 1 × 10 4 cells per well in white 96-well plates (Greiner Bio-one) and cultured in the astrocyte medium (DMEM, 10% FBS) for 7 days. The D90A MNX1+ MNs derived from SYP-Nluc reporter iPSC line were the plated at 1 × 10 4 cells per well on astrocytes and cultured in a nutrition-deficient medium (DMEM/F12, Neurobasal medium at 1:1, 1 × N2, 0.5 μM RA and 0.1 μM Compound E). For testing the compounds, Riluzole (50 μM, Torcris), Kenpaullone (5 μM, Tocris) and EphA inhibitor (50 μM, Calbiochem) were added in the medium. After co-culturing for 10 days, the Nluc activity was detected by Nano-Glo Luciferase Assay (Promega) according to the manufacturer’s instructions. Statistical analyses No statistical methods were used to predetermine sample sizes, but the samples sizes we used were consistent with those generally employed in the field. Comparisons between two groups were analysed by unpaired t -test with Welch’s correction. Multiple comparisons were analysed by one-way analysis of variance followed by Tukey’s multiple comparisons test. P <0.05 was considered to be statistically significant. Statistical processing was performed using the Microsoft Excel and GraphPad Prism Software. How to cite this article: Du, Z.W. et al. Generation and expansion of highly pure motor neuron progenitors from human pluripotent stem cells. Nat. Commun. 6:6626 doi: 10.1038/ncomms7626 (2015).